Mechanism for spectral break in cosmic ray proton spectrum of supernova remnant W44 Recent observations of supernova remnant W44 by the Fermi spacecraft observatory support the idea that the bulk of galactic cosmic rays is accelerated in such remnants by a Fermi mechanism, also known as diffusive shock acceleration. However, the W44 expands into weakly ionized dense gas, and so a significant revision of the mechanism is required. Here, we provide the necessary modifications and demonstrate that strong ion-neutral collisions in the remnant surrounding lead to the steepening of the energy spectrum of accelerated particles by exactly one power. The spectral break is caused by Alfven wave evanescence leading to the fractional particle losses. The gamma-ray spectrum generated in collisions of the accelerated protons with the ambient gas is calculated and successfully fitted to the Fermi Observatory data. The parent proton spectrum is best represented by a classical test particle power law ∝ E −2 , steepening to E −3 at E br ≈7 GeV due to deteriorated particle confinement. Ongoing direct observations of a number of galactic supernova remnants (SNRs) in the X- and gamma-ray bands supported by the radio, optical and ultraviolet data [1] , [2] seem to rapidly close in on the century long problem of the cosmic ray (CR) origin. Overall, the observations favour the diffusive shock acceleration (DSA, operating in SNR shocks) as a mechanism for the production of galactic CRs. However, there are at least two critical questions that observations pose to the theory. First, what exactly is the form of the spectrum that the theory predicts? Second, when do we really see the proton (that is, the primary CR component) emission and when do we see just a contaminating but radiatively more efficient electron component? Several decades of studies of the background galactic CRs, preceding direct observations (which became available only recently) demonstrated that already a simple test particle (TP) version of the DSA (leading to a power law ∝ E −2 particle energy distribution) reproduces the form of the energy spectrum reasonably well. It is possible, however, that a somewhat steeper power law would better accommodate the E −2.7 measured spectrum [3] , [4] (see also the Discussion), even though this difference can be attributed to CR propagation losses (also not completely certain). Nevertheless, the direct observations of emission coming from particles accelerated in SNR shocks often indicate significantly steeper than E −2 spectra [5] . Also the recent Fermi Large Area Telescope (LAT) observations of the SNR W44 suggest that the spectrum of the gamma-ray-producing protons is substantially steeper at high energies than the DSA predicts [6] . It should be noted that a similar discrepancy has already been found in the high-energy gamma-ray spectrum of the SNR RXJ 1713 measured by the CANGAROO [7] and HESS [5] atmospheric Cerenkov telescopes. The simple DSA prediction was even used as an argument against the hadronic origin of the gamma emission on the ground that if the high energy part of the spectrum was extrapolated (with the DSA index 2) to lower energies, the emission there would be unacceptably high, for example, see ref. 8 . Motivated by this inconsistency with the DSA theory in particular, we have previously published a suggestion of the mechanism for the spectral break [9] , which can resolve the discrepancies. We believe that a similar phenomenon is also applicable to the recent observations of the SNR W44. Here, we show that ion-neutral collisions in a molecular cloud adjacent to the remnant steepen the energy spectrum of accelerated particles. We calculate the gamma-ray spectrum resulting from the collisions of accelerated protons with the molecular cloud material and fit the result to the Fermi Observatory data. Mechanism for the spectral break The physics of the spectral break is very simple. When a SNR shock approaches a molecular cloud (MC) or a pre-supernova swept-up shell, confinement of accelerated particles generally deteriorates. Because of the particle interaction with magnetic turbulence, confinement requires scales similar to the particle gyroradius [10] , [11] . As long as the waves are in a strongly ionized (closer to the shock) medium they propagate freely in a broad frequency range at the Alfven speed V A = B /√4 πρ i with the frequencies ω = kV A . Here, k is the wave number (assumed parallel to the local field B ) and ρ i is the ion mass density. As long as the Alfven wave frequency is higher than the ion-neutral collision frequency v in , the waves are weakly damped. When, on the other hand, the ion-neutral collision frequency is higher (deeper into the cloud), neutrals are entrained by the oscillating plasma and the Alfven waves are also able to propagate, albeit with a factor √ ρ i / ρ 0 <1 lower speed, where ρ 0 is the neutral density. The propagation speed reduction occurs because every ion is now 'loaded' with ρ i / ρ 0 neutrals. In between these two regimes, Alfven waves are heavily damped and even disappear altogether for sufficiently small ρ i / ρ 0 <<0.1. The evanescence wave number range is then bounded by k 1 = v in /2 V A and k 2 =2√ ρ i / ρ 0 v in / V A . These phenomena have been studied in detail in refs 12 , 13 , and specifically in the context of the DSA in refs 14 , 15 , 16 . Now, we turn to their impact on the particle confinement and emissivity. In the frame work of a quasilinear wave-particle interaction, the wave number k is approximately related to the parallel (to the magnetic field) component of the particle momentum p || by the cyclotron resonance condition kp || / m =± ω c , where the (non-relativistic) gyro-frequency ω c = eB / mc . 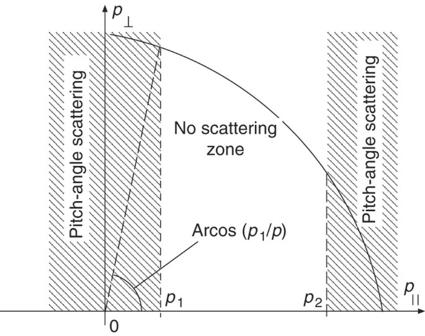Figure 1: Momentum space of accelerated protons. Particle scattering zones on the (p||,p⊥) plane of momentum space. Particles in the stripesp1<|p|||<p2are not scattered by waves (see text). Therefore, particles from the domains |p|||>p2maintain their propagation direction and promptly escape from the dense gas region. Therefore, the frequency range where the waves cannot propagate may be conveniently translated into the parallel momentum range with That a spectral break must form at the photon energy corresponding to the particle momentum p = p 1 = p br , can be readily understood from Figure 1 . The 'dead zones' p 1 <| p || | <p 2 imply that particles with | p || |> p 1 do not turn around (while moving along the magnetic field) and escape from the region of CR-dense gas collisions at a p || / p fraction of the speed of light. This happens in the region of enhanced gamma radiation. Therefore, an initially isotropic distribution of accelerated particles fills only a slab in momentum space | p || |< p 1 and becomes highly anisotropic (a 'pancake' distribution). What matters for the integral emission, however, is a locally isotropic component f̄ of this new proton distribution. It can be introduced by re-averaging the 'pancake' (| p || |< p 1 ) distribution in pitch angle, d μ , and is readily obtained assuming that particles remaining in the dense gas (those with | p || |< p 1 ) maintain their isotropic pitch-angle distribution, that is where f 0 ( p ) is the initial (isotropic) distribution function and μ is the cosine of the pitch angle (see Fig. 1 ), μ 1 =min{ p 1 / p ,1}. Thus, the slope of the particle momentum distribution becomes steeper by exactly one power above p = p 1 ≡ p br . In particular, any power law distribution ∝ p − q , on entering an MC, turns into p − q −1 at p ≥ p br , and preserves its form at p < p br . Figure 1: Momentum space of accelerated protons. Particle scattering zones on the ( p || , p ⊥ ) plane of momentum space. Particles in the stripes p 1 <| p || |< p 2 are not scattered by waves (see text). Therefore, particles from the domains | p || |> p 2 maintain their propagation direction and promptly escape from the dense gas region. Full size image Now the question is whether particle escape from the MC can quench the acceleration process itself. In principle it can, as the particles from the interval | p || |< p 1 cannot return to the shock and continue acceleration. Instead, by slowly leaking to the part of the momentum space with | p || |> p 1 , they should ultimately escape as well. This would certainly be the case if the MC were filling the entire shock precursor. However, MCs are known to be clumpy [17] , [18] , [19] , and may fill only a small fraction of the precursor. In this case, the acceleration process continues almost unimpeded, the accelerated protons illuminate the 'cloudlets' and make them visible in γ-rays becasue of the high-density target material. Break momentum Although the one power spectral break in the pitch-angle averaged particle distribution seems to be a robust environmental signature of a weakly ionized medium into which the accelerated particles propagate, the break momentum remains uncertain. According to equation (2), p br (≡ p 1 ) depends on the magnetic field strength and ion density as well as on the frequency of ion-neutral collisions, v in = n 0 〈 σV 〉. Here, 〈 σV 〉 is the product of the collision cross-section and collision velocity averaged over the thermal distribution. Using an approximation from (refs 15 , 20 ) for 〈 σV 〉, p br can be estimated as Here, the gas temperature T 4 is measured in the units of 10 4 K, magnetic field B μ -in microgauss, n 0 and n i (number densities corresponding to the neutral/ion mass densities ρ 0 and ρ i ) -in cm −3 . Note that the numerical coefficient in the last expression may vary depending on the average ion and neutral masses and can be higher by a factor of a few for typical MC conditions [12] , [21] than the estimate in equation (4) suggests. The remaining quantities in the last formula are also known too poorly to make an accurate independent prediction of the position of the break in the gamma-ray emission region. Those are the regions near the blast wave where complicated physical processes unfold. They include particle acceleration, strong magnetohydrodynamic (MHD) turbulence (driven by particles and their interaction with ambient gas inhomogeneities), gas ionization by shock generated ultraviolet photons, turbulent plasma heating and even evaporation of magnetic cloudlets [20] , [22] , [23] . Also important may be the ionization by the low-energy CRs accelerated at the blast wave. However, as their diffusion length is shorter than that of the particles with p ≳ p br , we may assume that they do not reach the MC. Preionization by the ultraviolet photons can also be ignored for the column density N >10 9 cm −2 ahead of the shock beyond which they are absorbed [24] . The authors of the (ref. 24 ), using the earlier data from ref. 25 , have also analysed the parameters involved in equation (4) and found the above estimate of p br to be in a good agreement with the spectral break position measured by the Fermi LAT. Nevertheless, we may run the argument in reverse and use the Fermi observations [6] of the gamma-ray spectrum of SNR W44 to determine the break momentum in the parent particle spectrum and constrain the parameters in equation (4). Once we also know the amount of the slope variation Δ q , we can calculate the full spectrum up to the cutoff energy. Particle spectra To calculate the particle spectra, we need to determine the degree of nonlinear (NL) modification of the shock structure. In principle, it can be calculated consistently, given the shock parameters and the particle maximum momentum, p max . In the case of a broken spectrum, p br has the role of p max , as this is the momentum where the dominant contribution to the pressure of accelerated particles comes from, thus setting the scale of the modified shock precursor. Note that in the conventional NL acceleration theory, the cutoff momentum p max has this role, because the NL spectra are sufficiently flat so as to make the pressure diverge with momentum. The break in the photon spectrum is observed at about 2 GeV, which places the break on the proton distribution at about p br ⋍ 7 GeV/c (ref. 6 ). For the strength of the break Δ q =1, the spectrum above it is clearly pressure converging, and we perform the calculation of the shock structure and the spectrum using this break momentum as the point of the maximum in the CR partial pressure. Once this point is set, we can use an analytic approach for a stationary NL acceleration problem using p br as an input parameter. Apart from p br , the NL solution depends on a number of other parameters, such as the injection rate of thermal particles into acceleration, Mach number, the precursor heating rate and the shock velocity V s . Of these parameters, only the latter is known accurately, V s ≈300 km s −1 , the other parameters are still difficult to ascertain. Fortunately, in sufficiently strong shocks the solution generally tends to either stay close to the TP solution (leaving the shock structure only weakly modified) or else it transitions to a strongly modified NL-solution regime. The TP regime typically establishes in cases of moderate Mach numbers, low injection rates and low p max (now p br ), whereas the NL regime is unavoidable in the opposite part of the parameter space. In the TP regime, the spectrum is close to a power law with the spectral index 2 throughout the supra-thermal energy range. In the NL regime, however, the spectrum develops a concave form, starting from a softer spectrum at the injection energy, with the index q ⋍ ( r s +2)/( r s −1)>2, where r s <4 is the sub-shock compression ratio. Then it hardens, primarily in the region p ∼ mc, where both the partial pressure and diffusivity of protons change their momentum scaling. The slope reaches its minimum at the cutoff (break) energy, which, depending on the degree of nonlinearity, can be as low as 1.5 or even somewhat lower if the cutoff is abrupt. The question now is into which of these two categories the W44 spectrum falls? Generally, in cases of low maximum (or, equivalently, low spectral break p br ≲ 10) momentum, the shock modification is weak, so the spectrum is more likely to be in the only slightly NL, almost TP regime. On the other hand, there is a putative indication from the electron radio emission that their spectrum may be close to q e ≈1.75, which could be the signature of a moderately NL acceleration process. It should be remembered, however, that this is a global index across the W44 remnant. There are resolved bright filaments where a canonical α =−0.5 spectrum, corresponding precisely to the TP parent electron spectrum with q e =2 is observed [26] . Moreover, there are regions with the positive indices α ≲ 0.4, which cannot be indicative of a DSA process without corrections for subsequent spectral transformations such as an absorption by thermal electrons [26] . These regions can very well contribute to the overall spectral hardening discussed above, mimicking the acceleration nonlinearity. Finally, secondary electrons give rise to the flattening of the radio spectrum as well [24] . If the accelerated protons and electrons respond to the turbulence in a similar manner, which is almost certainly the case in the ultra-relativistic regime, their spectra should have similar slopes in that region (as long as the synchrotron losses are ignorable). In using the electron radio spectrum as a probe for the level of acceleration nonlinearity, the following two relations are useful. First, there is a relation between the electron energy and the radio frequency v MHz =4.6· B μ E 2 GeV . The second relation, q e =1−2 α , links the spectral index of radio emission α (assuming the radio flux ∝ v α ) and the spectral index of the parent electrons q e (assuming their energy spectrum ∝ E − qe ). Once the global radio spectral index of W44, α ⋍ −0.37 (ref. 26 ) is generated by freshly accelerated electrons in the frequency range 74< v <10,700 MHz, the electrons should maintain their modified spectrum over the energy range spanning more than one order of magnitude. For example, assuming B μ ⋍ 70 (ref. 6 ), one sees that electrons must maintain an index q e ≈1.75 between 0.46< E <5.8 GeV. Although the upper bound is acceptable given the spectral break proton energy inferred from the super GeV emission measured by the Fermi LAT, the lower end is rather uncomfortable, as the NL modification of both protons and electrons with the Bohm (or other similar for protons and electrons turbulent diffusivities) starts (slowly) only at the proton rest energy. 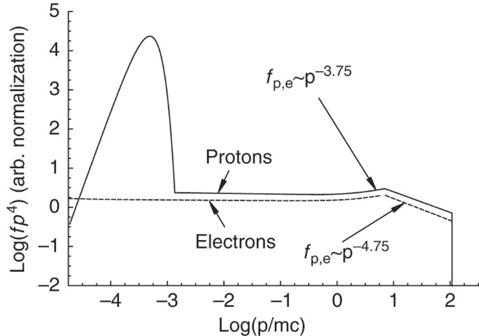Figure 2: Spectra of accelerated protons and electrons. Both particle distributions are calculated for a weakly modified shock and are shown in momentum normalization (f(p) is steeper by two powers than the spectra in energy normalization, used in the text). Both spectra are multiplied byp4, so that the test particle distribution is flat. Shock parameters: acoustic Mach numberM=30, shock velocityVs/c=10−3, the break momentumpbr⋍7 mc. Shock pre-compression (flow compression across the CR precursor)R=1.8, injection parameterv⋍0.1 (defined asv=(4π/3)(mc2/ρVs2)(pinj/mc)4f(pinj), withρandVsbeing the ambient gas density and the shock speed, respectively); injection momentumpinj/mc⋍1.4×10−3 The calculated NL spectra are shown in Figure 2 for the both species. At and below 1 GeV, the electron spectrum is very close to the TP solution, q e ≈2 even though the proton spectrum may be somewhat steeper there, as we mentioned above. Figure 2: Spectra of accelerated protons and electrons. Both particle distributions are calculated for a weakly modified shock and are shown in momentum normalization ( f ( p ) is steeper by two powers than the spectra in energy normalization, used in the text). Both spectra are multiplied by p 4 , so that the test particle distribution is flat. Shock parameters: acoustic Mach number M =30, shock velocity V s /c=10 −3 , the break momentum p br ⋍ 7 mc. Shock pre-compression (flow compression across the CR precursor) R =1.8, injection parameter v ⋍ 0.1 (defined as v =(4 π /3)(mc 2 / ρV s 2 )( p inj /mc) 4 f( p inj ), with ρ and V s being the ambient gas density and the shock speed, respectively); injection momentum p inj /mc ⋍ 1.4×10 −3 Full size image Photon spectra The above considerations somewhat weaken the radio data as a probe for the slope of the electron and (more importantly) for the proton spectrum. Therefore, the exact degree of nonlinearity of the acceleration remains unknown and we consider both the TP and weakly NL regimes in our calculations of the photon spectra, generated in p − p collisions. 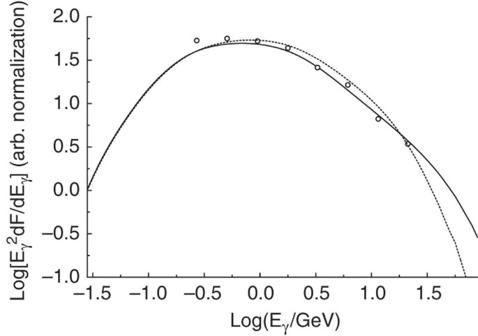Figure 3: Gamma-radiation spectra. Photon spectra resulting fromπ0decay and calculated for two different parent proton spectra compared against the Fermi data (open circles). Solid line: a TP acceleration regime with the spectral indexq=2 below the break andq=3 above the break atpbr=7 GeV/c. Dashed line: a moderately nonlinear acceleration regime corresponding to the spectrum shown inFigure 2(q⋍1.75 andq⋍2.75 below and above the break, respectively). Cut-offs are placed at 300 GeV for TP- and 100 GeV for NL-spectrum. The results are shown in Figure 3 . The best fit to the Fermi data is provided by a TP energy distribution ( ∝ E −2 ) below p br ⋍ 7 GeV/c with the spectrum steepening by exactly one power above it. Note that the small deviation of the computed spectrum from the lowest energy Fermi- point may also be corrected by including the Bremsstrahlung of the secondary electrons [24] . The spectrum steepening is perfectly consistent with the proton partial escape described above (with no parameters involved) and shown in Figure 1 . For comparison, a weakly NL spectrum, shown in Figure 2 , is also used for these calculations (dashed line in Fig. 3 ), but its fit would require a stronger break (Δ q >1) or a low momentum cutoff, Figure 3 , that is, at least one additional free parameter. Figure 3: Gamma-radiation spectra. Photon spectra resulting from π 0 decay and calculated for two different parent proton spectra compared against the Fermi data (open circles). Solid line: a TP acceleration regime with the spectral index q =2 below the break and q =3 above the break at p br =7 GeV/c. Dashed line: a moderately nonlinear acceleration regime corresponding to the spectrum shown in Figure 2 ( q ⋍ 1.75 and q ⋍ 2.75 below and above the break, respectively). Cut-offs are placed at 300 GeV for TP- and 100 GeV for NL-spectrum. Full size image To summarize the results, the previously suggested mechanism for a break on the spectrum of shock accelerated protons [9] is found consistent with the recent [6] Fermi LAT observations of the SNR W44. The observed gamma-ray spectrum most likely results from the decay of π 0 -mesons, which are born in p − p collisions of shock accelerated protons with an ambient dense gas. The parent proton spectrum is best represented by a classical TP power law ∝ E −2 , steepening to E −3 at E br ≈7 GeV because of deteriorated particle confinement caused by the ion-neutral collisions and the resultant Alfven wave evanescence. The position of the break momentum in the particle spectrum may be estimated using equation (4), or conversely, the combination of parameters involved in this estimate can be inferred from the measured break momentum. The cutoff momentum is not constrained in this scenario. An alternative explanation, based on a different mechanism of the break, associated with the change of the particle transport in the CR shock precursor [27] is also possible, but is less definitive in the spectrum slope variation Δ q across the break (see also ref. 24 for the most recent alternative suggestions). In addition, the mechanism described in (ref. 27 ) would imply a considerable nonlinearity, that is, a stronger CR shock precursor than it seems appropriate for the observed low break momentum. Still alternatively, assuming our 'environmental' break mechanism is at work, that is, Δ q=1 , but the shock structure appreciably modified, we arrive at the E −1.75 spectrum below the break (as the radio observations suggest for the electrons), and E −2.75 above the break. A fit to the data is marginally possible, but it would require a relatively low cutoff momentum at about 100 GeV/c. This possibility may be supported or ruled out once the data (upper limit) around this energy become available. The most robust and attractive aspect of the suggested mechanism for the spectral break is the exact Δ q =1 variation of the spectral index. Indeed, this change in the spectral slope is due to truncation of the particle momentum phase space and does not depend on any parameters. In a combination with the TP regime operating below the break, which is consistent with the low value of the break momentum, it provides a very good fit to the Fermi LAT data. Of three physically different types of spectral breaks suggested earlier [9] , [27] , [28] , the current 'environmental' mechanism appears to be plausible in situations in which dense target gas is present, as required for efficient π 0 production. In a more general context, a spectral break is a natural resolution of the well-known but puzzling trend of the NL (that is, supposedly improved) DSA theory to develop spectra, which are even harder than the simple TP spectra, thus encountering more difficulties while accommodating the bulk of observations [3] , [4] . Such a spectrum—that is, diverging in energy—exhausts the shock energy available for the acceleration as the cutoff momentum grows. Note, that the spectrum of the RX J1713.7-3946 (ref. 5 ) is also consistent with the same break mechanism, but with p br ∼ 10 3 GeV/c and with naturally stronger acceleration nonlinearity [9] . However, it is difficult to make the case for hadronic origin of the gamma-ray emission of the RX J1713.7-3946 (refs 5 , 29 , 30 ). The fundamental role of the W44 for the problem of CR origin is that this particular remnant seems to rule out contaminating electron emission due to Bremsstrahlung and the inverse Compton scattering [6] , [24] , thus favouring the hadronic origin of the gamma emission. Acceleration model and proton spectrum Methods of calculation of the accelerated particle spectra, including the particle back-reaction on the shock structure, are now well developed. We use the diffusion–convection equation for describing the distribution of high-energy particles (CRs). To include the back-reaction, three further relations are used in a quasi-stationary acceleration regime. These are the conservation of mass and momentum fluxes in the smooth part of the shock transition (so-called CR-precursor) and the Rankine–Hugoniot relation for the shock compression at the gaseous discontinuity (sub-shock). The complete system of equations is then reduced to one NL integral equation [31] . This equation is solved numerically and the results are shown in Figure 1 . The above method of calculation of the parent particle spectra is shown to be in excellent agreement [32] with numerical simulations [33] , [34] , as well as with other semi-analytic approaches [35] . Gamma-ray emission spectrum Once the parent proton spectrum is obtained, we calculate the π 0 production rate and the gamma-ray emissivity. In so doing, we adopt numerical recipe described in detail in refs 36 , 37 . The physical processes behind these calculations are [38] : collisions of accelerated protons with the protons of the ambient gas resulting in the following spectrum of π 0 -mesons: where, N pg is the number density of protons in the gas, dσ / dE π is the differential cross-section for the π 0 production in collisions between accelerated protons of energy E p and gas protons, J p is the flux of accelerated protons, E π is the energy of π 0 mesons; and decay of π 0 resulting in the gamma emission spectrum where m π is the pion rest mass. How to cite this article : Malkov, M. A. et al . Mechanism for spectral break in cosmic ray proton spectrum of Supernova remnant W44. Nat. Commun. 2:194 doi: 10.1038/ncomms/1195 (2011).